Integrated circuit-based electrochemical sensor for spatially resolved detection of redox-active metabolites in biofilms Despite advances in monitoring spatiotemporal expression patterns of genes and proteins with fluorescent probes, direct detection of metabolites and small molecules remains challenging. A technique for spatially resolved detection of small molecules would benefit the study of redox-active metabolites that are produced by microbial biofilms and can affect their development. Here we present an integrated circuit-based electrochemical sensing platform featuring an array of working electrodes and parallel potentiostat channels. ‘Images’ over a 3.25 × 0.9 mm 2 area can be captured with a diffusion-limited spatial resolution of 750 μm. We demonstrate that square wave voltammetry can be used to detect, identify and quantify (for concentrations as low as 2.6 μM) four distinct redox-active metabolites called phenazines. We characterize phenazine production in both wild-type and mutant Pseudomonas aeruginosa PA14 colony biofilms, and find correlations with fluorescent reporter imaging of phenazine biosynthetic gene expression. For studying biological systems, optical microscopy techniques remain paramount. Using photons affords the advantage of relatively non-invasive interaction with the biological system under study [1] . In such techniques, the solid-state interface to the biological system is usually a complementary metal-oxide-semiconductor (CMOS) or charge-coupled device imager. The use of such wide-field imagers allows massively parallel measurement of many optical reporters within a field of view. In this context, protein-based fluorescent reporters are routinely used for in situ observation of transcriptional dynamics [2] . These constructs enable localization of gene or protein expression within cellular communities and multicellular organisms and have greatly expanded our understanding of diverse biological systems, as development is dictated by the spatial and temporal control of protein expression. However, the fluorescent reporter technique cannot be used to directly detect critical components of physiology such as primary metabolism and signalling factors that influence these changes in expression. Direct detection of small molecules can be facilitated by techniques employing direct transduction to electrons, without using photons as an intermediary. Approaches to electronic transduction include field-effect techniques, in which charge is used to modulate the current in a semiconductor [3] , [4] , [5] , and electrochemical techniques, in which oxidation or reduction of electrochemically active molecules is measured [6] . A scanning system can be employed with a single transducer, but achieving the large-scale parallelism possible with wide-field optical imaging requires integrating these transducers, as well as front-end amplifiers and multiplexing circuitry, onto an active CMOS chip. An application uniquely suited to electrochemical, rather than photonic, transduction that would benefit from CMOS electrochemical sensory arrays is direct imaging of redox-active signalling molecules in biofilms. The opportunistic pathogen P. aeruginosa PA14 produces redox-active metabolites called phenazines, which vary in structure and chemical properties [7] , [8] and have individualized, drastic effects on community behaviour in colony biofilms grown for several days on the surface of an agar plate [9] , [10] , [11] . Phenazine-null mutants form colonies that spread over the surface of the agar plate and exhibit highly wrinkled structures. Production of phenazines prevents spreading and wrinkling, leading to more constrained and smoother morphologies ( Fig. 1a ). At least four different phenazines are produced by P. aeruginosa PA14: phenazine-1-carboxylic acid (PCA), phenazine-1-carboxamide (PCN), pyocyanin (PYO) and 5-methylphenazine-1-carboxylic acid (5-MCA). PCA is produced from chorismate by the phenazine biosynthetic enzymes PhzA-G [12] . PCA, in turn, is converted to PCN in a reaction catalysed by the enzyme PhzH. PCA is also methylated by the enzyme PhzM to produce 5-MCA, which can be further converted into PYO by the monooxygenase PhzS ( Fig. 1b ). The different functional groups surrounding the core phenazine structure affect the chemical properties and redox potentials of individual derivatives ( Fig. 1c ) [13] . To study the contributions of phenazines to colony development, a better understanding of their spatiotemporal production pattern is crucial. However, attempts to detect phenazines and other similar classes of compounds by their own fluorescence [14] or using fluorescent dyes [15] are limited by nonspecific reactivity and poor imaging sensitivity. 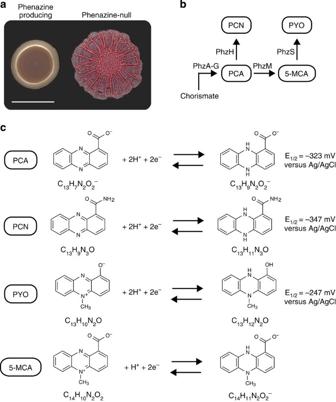Figure 1: Phenazines and their properties. (a) Phenazines affect morphogenesis ofP. aeruginosaPA14 colony biofilms9,11. Phenazine producing strain=BigBlue; phenazine-null strain=Δphz(seeSupplementary Table 1). Colony biofilms are imaged after 3 days of development. Scale bar, 1 cm. (b) Phenazine biosynthetic pathway inP. aeruginosa. Arrows are labelled with the enzymes catalysing the various conversion reactions12. PCA, phenazine-1-carboxylic acid; PCN, phenazine-1-carboxamide; PYO, pyocyanin; 5-MCA, 5-methylphenazine-1-carboxylic acid. (c) Phenazine redox reactions, with redox potentials shown for pH=7 (ref.13). Figure 1: Phenazines and their properties. ( a ) Phenazines affect morphogenesis of P. aeruginosa PA14 colony biofilms [9] , [11] . Phenazine producing strain=BigBlue; phenazine-null strain=Δ phz (see Supplementary Table 1 ). Colony biofilms are imaged after 3 days of development. Scale bar, 1 cm. ( b ) Phenazine biosynthetic pathway in P. aeruginosa . Arrows are labelled with the enzymes catalysing the various conversion reactions [12] . PCA, phenazine-1-carboxylic acid; PCN, phenazine-1-carboxamide; PYO, pyocyanin; 5-MCA, 5-methylphenazine-1-carboxylic acid. ( c ) Phenazine redox reactions, with redox potentials shown for pH=7 (ref. 13 ). Full size image A few studies have employed electrochemical techniques for detecting and quantifying phenazines produced by P. aeruginosa PA14 liquid cultures [16] , [17] , [18] , [19] . Scanning electrochemical microscopy has been used to study phenazines at the surface of biofilms in a spatially resolved manner [20] , but without the ability to quantify concentration or to simultaneously detect multiple redox-active species. In contrast, the electrochemical sensor array chip developed here can directly quantify in a spatially resolved manner the concentrations of multiple phenazines released by biofilms into the underlying agar. The chip is capable of capturing a 60-pixel image in only 36 s at sensitivities down to 2.6 μM. Phenazines are particularly well-suited for this imaging technique because of their strong redox activities and distinct redox signatures. In this study, we electrochemically characterize four phenazines produced by P. aeruginosa PA14 and use our CMOS electrochemical sensing platform for spatially resolved detection and quantification of multiple phenazines in both wild-type (WT) and mutant P. aeruginosa PA14 biofilms. We also correlate these findings with fluorescent reporter imaging of phenazine biosynthetic gene expression. Integrated circuit sensing platform These studies use a custom-designed integrated circuit (IC), a 5 × 5 mm 2 chip fabricated in a 0.25-μm CMOS process. The IC features an integrated control amplifier at the core of a potentiostat capable of establishing on-chip electrochemical cells with an array of 60 100 × 100-μm 2 thin film gold working electrodes, as well as five measurement channels containing integrated transimpedance amplifiers (TIAs) each multiplexed to 12 working electrodes. The electrochemically measured concentrations of phenazines at individual electrodes in the on-chip array can serve as a spatially resolved image of phenazine production by the colony. A diagram and image of the chip are shown in Fig. 2a,b , respectively. 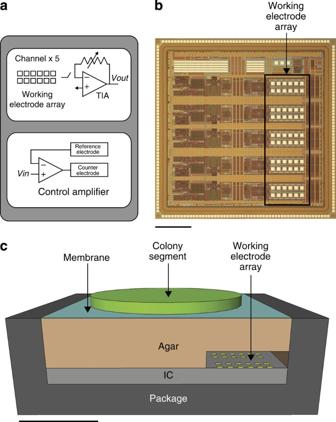Figure 2: On-chip colony biofilm experimental setup. (a) Block diagram of the integrated circuit (IC). (b) Optical micrograph of the IC, with the working electrode array highlighted. Scale bar, 1 mm. (c) Schematic of the experimental setup, including the colony, IC and agar interface membrane. Scale bar, 1 mm. Figure 2: On-chip colony biofilm experimental setup. ( a ) Block diagram of the integrated circuit (IC). ( b ) Optical micrograph of the IC, with the working electrode array highlighted. Scale bar, 1 mm. ( c ) Schematic of the experimental setup, including the colony, IC and agar interface membrane. Scale bar, 1 mm. Full size image Rather than placing the IC in direct contact with the top of the colony, which will disturb the colony morphology, we access phenazines from the bottom of the colony by interposing between the colony and the IC a layer of agar through which phenazines diffuse and are detected. This agar layer must be thin (in our case, approximately 1 mm), as this thickness directly determines the spatial resolution achievable by the array. As bacterial colonies do not produce pronounced structures when grown on agar layers that are this thin, we grow P. aeruginosa PA14 colonies on track-etched membranes positioned on top of >5-mm thick agar layers. These membranes have a pore size of 0.4 μm, which allows passage of nutrients and phenazines and does not interfere with colony development. Before each measurement, we transfer the colony and membrane from the thick agar layer to a thin l-mm agar layer on the IC ( Fig. 2c ). Electrochemical characterization of phenazines Although the chip supports generalized potentiostatic analysis (including electrochemical impedance spectroscopy and cyclic voltammetry), we use square wave voltammetry (SWV) to characterize phenazine production. Each current-versus-voltage voltammogram is characterized by a current peak. The voltage at which this current peak occurs is dependent on the redox potential of the measured species and the magnitude of the peak is proportional to the species’ concentration. Accurate measurement of Faradaic peak currents (and hence concentrations) is difficult in traditional cyclic voltammetry because the Faradaic response is superimposed on an imprecisely known non-Faradaic charging current. In SWV, current responses to successive forward and reverse voltage steps are subtracted, removing the non-Faradaic current components [21] . To demonstrate the ability to distinguish phenazines electrochemically, P. aeruginosa PA14 colonies are grown on a solid medium containing 1% agar and 1% tryptone. Secreted phenazines are extracted from the agar into phosphate-buffered saline after 1 day of colony growth. In addition to analysing colonies of WT P. aeruginosa PA14, whose agar extract contains a complex mixture of phenazines, we use mutant colonies, each of which lacks specific phenazine biosynthetic enzymes and, therefore, only produces a subset of the phenazines discussed above (see Supplementary Tables 1 and 2 ). This allows us to analyse agar extracts containing simpler mixtures of phenazines. These mutants include Δ phz , which produces no phenazines; Δ phzHM , which produces only PCA; Δ phzHS , which produces PCA and 5-MCA; Δ phzH , which produces PCA, 5-MCA and PYO; and Δ phzMS , which produces PCA and PCN. High-performance liquid chromatography is used to confirm that each mutant produces the expected phenazines ( Fig. 3a ), except for 5-MCA, which we cannot detect using this method. 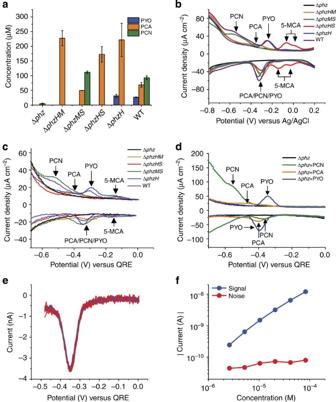Figure 3: Electrochemical characterization of phenazines. (a) Average concentration, quantified spectrophotometrically, of high-performance liquid chromatography (HPLC)-separated phenazines extracted from agar on which colonies of variousP. aeruginosastrains grew for 1 day. The average is taken from three samples, with error bars representing the standard deviation among the three samples. (b) Commercial potentiostat-generated square wave voltammograms of extracts from agar on which colonies ofP. aeruginosaPA14 (wild type, WT) and various PA14 mutants grew for 1 day. (c) Integrated circuit (IC)-generated square wave voltammograms of phenazines secreted into agar by variousP. aeruginosaPA14 mutant colonies placed onto the IC. Voltammograms from multiple measurements are averaged and the results shifted vertically to a common baseline to facilitate comparison. (d) IC-generated square wave voltammograms of extract from agar on which Δphzcolonies grew for 1 day, with added synthetic/purified phenazines. Voltammograms from multiple measurements are averaged. (e) An example set of baseline-subtracted, negative-to-positive square wave voltammograms at 21 μM, used for the signal and noise characterization. A single square wave voltammogram is shown in blue, whereas 19 others are shown in red. (f) Results from on-chip square wave voltammetry (SWV) of multiple concentrations of PYO solutions in agar. Signal level represents the peak current from one square wave voltammogram. Signal levels are shown after subtraction of theyaxis intercept of a linear fit to measured signal levels, which represents the current at 0 μM. Noise level represents the standard deviation in peak currents from 20 averaged square wave voltammograms. PCA, phenazine-1-carboxylic acid; PCN, phenazine-1-carboxamide; PYO, pyocyanin; QRE, quasireference electrode; 5-MCA, 5-methylphenazine-1-carboxylic acid or a derivative thereof. In SWV figures, upper traces are for positive-to-negative and lower traces are for negative-to-positive. Phenazines responsible for peaks are labelled above those peaks. Figure 3: Electrochemical characterization of phenazines. ( a ) Average concentration, quantified spectrophotometrically, of high-performance liquid chromatography (HPLC)-separated phenazines extracted from agar on which colonies of various P. aeruginosa strains grew for 1 day. The average is taken from three samples, with error bars representing the standard deviation among the three samples. ( b ) Commercial potentiostat-generated square wave voltammograms of extracts from agar on which colonies of P. aeruginosa PA14 (wild type, WT) and various PA14 mutants grew for 1 day. ( c ) Integrated circuit (IC)-generated square wave voltammograms of phenazines secreted into agar by various P. aeruginosa PA14 mutant colonies placed onto the IC. Voltammograms from multiple measurements are averaged and the results shifted vertically to a common baseline to facilitate comparison. ( d ) IC-generated square wave voltammograms of extract from agar on which Δ phz colonies grew for 1 day, with added synthetic/purified phenazines. Voltammograms from multiple measurements are averaged. ( e ) An example set of baseline-subtracted, negative-to-positive square wave voltammograms at 21 μM, used for the signal and noise characterization. A single square wave voltammogram is shown in blue, whereas 19 others are shown in red. ( f ) Results from on-chip square wave voltammetry (SWV) of multiple concentrations of PYO solutions in agar. Signal level represents the peak current from one square wave voltammogram. Signal levels are shown after subtraction of the y axis intercept of a linear fit to measured signal levels, which represents the current at 0 μM. Noise level represents the standard deviation in peak currents from 20 averaged square wave voltammograms. PCA, phenazine-1-carboxylic acid; PCN, phenazine-1-carboxamide; PYO, pyocyanin; QRE, quasireference electrode; 5-MCA, 5-methylphenazine-1-carboxylic acid or a derivative thereof. In SWV figures, upper traces are for positive-to-negative and lower traces are for negative-to-positive. Phenazines responsible for peaks are labelled above those peaks. Full size image Phenazines from colonies are first subjected to SWV electrochemical analysis with a commercial potentiostat in a standard three-electrode macroelectrode configuration and then with the integrated IC potentiostat. For the IC platform, a Ag/AgCl quasireference electrode (QRE) is used. SWV is performed with inputs proceeding from negative to positive voltages (‘negative-to-positive SWV’) and repeated with inputs proceeding from positive to negative voltages (‘positive-to-negative SWV’) on agar extracts from mutant colonies ( Fig. 3b ). For the settings used here (see Methods), there are no peaks in square wave voltammograms from the Δ phz mutant, which differs from the WT only in its lack of phenazines. This finding indicates that all peaks in square wave voltammograms from phenazine-producing mutants must be due to phenazines, and not other classes of redox-active metabolites. We then compare the square wave voltammograms of extracts from mutant strains that differ in the production of only one phenazine. The appearance of a new current peak allows us to determine the electrochemical signature of the differing phenazine. We find the following SWV signatures for each phenazine: for PCA, −400 mV peak versus Ag/AgCl on positive-to-negative SWV and −300 mV peak on negative-to-positive SWV; for PYO, −250 mV peak on positive-to-negative SWV and −330 mV peak on negative-to-positive SWV; for PCN, −500 mV peak on positive-to-negative SWV and −330 mV peak on negative-to-positive SWV; and for 5-MCA, −70 mV peak on positive-to-negative SWV and −140 mV peak on negative-to-positive SWV. We should note that 5-MCA is predicted to be highly reactive [22] and therefore we cannot exclude that a 5-MCA derivative is present [23] . Indeed, the two peaks may indicate the presence of two compounds. For simplicity, we refer to the compounds responsible for peaks in this voltage range as ‘5-MCA’. The observed asymmetry between positive-to-negative and negative-to-positive voltammograms is not affected significantly by frequency (see Supplementary Fig. 1 ). Other studies have observed similar deviations from ideal Nernstian conditions at pH greater than 8 (ref. 13 ). We have found that performing both positive-to-negative and negative-to-positive SWV is not usually necessary. For distinguishing one phenazine in the presence of others, positive-to-negative SWV is used, because the peaks do not overlap as they do in negative-to-positive SWV. For analysing solutions containing just one phenazine, it may be preferable to use negative-to-positive SWV, in which peaks are more pronounced. After characterizing phenazines with standard instrumentation, we can study phenazines with the IC. All subsequent measurements we report are performed on the IC platform. Rather than extracting phenazines from agar into a solution as is done above for the commercial potentiostat experiments, we are able to place WT and mutant colony biofilms onto the IC and immediately analyse the secreted phenazines ( Fig. 3c ). Phenazine signatures from these experiments match the results of Fig. 3b . As a final confirmation experiment, we inject into agar extract from the Δ phz mutant, which lacks all phenazines, synthetic PYO (10 μM), synthetic PCA (300 μM) and PCN (3 mM) purified from P. aeruginosa PA14 liquid culture. (Due to the unavailability of purified or synthetic 5-MCA, we cannot perform this analysis for 5-MCA.) The on-chip square wave voltammograms ( Fig. 3d ) confirm the electrochemical signatures determined for endogenous phenazines ( Fig 3b,c ). (See Supplementary Fig. 2 for the voltammograms generated from the commercial potentiostat for synthetic phenazines.) The peak current value for a SWV peak is linearly related to the concentration of the redox species contributing to that peak [21] . For the case of PYO, we measure 20 negative-to-positive square wave voltammograms at various concentrations. To calculate signal level at a given concentration, we measure the peak current value on a single square wave voltammogram, and to calculate noise level, we measure the standard deviation of the peak currents on all 20 square wave voltammograms. An example of 20 square wave voltammograms for PYO at 21 μM is shown in Fig. 3e . Figure 3f shows the signal and noise levels for PYO in agar titrated down to 2.6 μM. At 2.6 μM, the signal-to-noise ratio (SNR) is approximately 5.5. The noise level is largely determined by flicker noise from the IC amplifiers and thermal noise from the feedback resistor network (see Supplementary Figs 3 and 4 and Supplementary Methods ). Characterization of phenazine diffusion Phenazines secreted by a colony biofilm diffuse both vertically and horizontally through the thin agar layer used to interface the biofilm to the measurement array. A longer delay between transferring the colony and performing the measurement allows for more phenazines to vertically diffuse to the sensing electrodes and, therefore, improves SNR, but longer diffusion times also allow horizontal diffusion to degrade the spatial resolution of the sensing platform. To estimate the diffusion coefficient of phenazines in agar, we perform a measurement in which a PYO-soaked membrane is placed above only a portion of the chip, as shown in Fig. 4a , and the PYO concentration is monitored over time at two electrodes, one directly below the membrane and one approximately 125 μm away from the membrane ( Fig. 4a ). In addition, we simulate this system using a three-dimensional diffusion model across a 4 × 4 × 0.9 mm 3 agar block with a constant concentration of PYO maintained at the top surface of a portion of the block ( Fig. 4b ). The concentration at the bottom surface of the block, representing what is presented for analysis to the measurement array, is simulated as a function of time ( Fig. 4c ). A good fit between the experimental and simulated data is found for a diffusion constant of 0.5 × 10 −9 m 2 s −1 for PYO in agar and concentration maintained at a constant 71 μM at the top surface of the agar ( Fig. 4d ). It is expected that comparable diffusion coefficients apply for other phenazines. 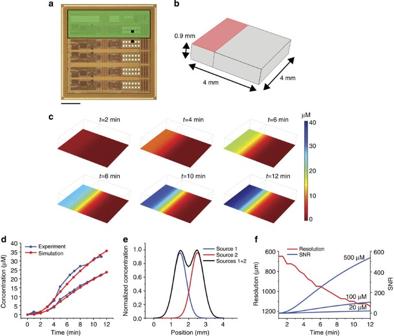Figure 4: Characterization of phenazine diffusion. (a) Experimental schematic for on-chip diffusion characterization. The pyocyanin (PYO)-soaked piece of membrane is shown in green, whereas the two probed electrodes are highlighted in black. Scale bar, 1 mm. (b) Simulation model of the experiment, consisting of a 4 × 4 × 0.9 mm3block with a constant 71 μM concentration at the blue surface. (c) Simulation results, showing concentration at the bottom surface of the block. (d) Experimental concentration-versus-diffusion time results at the two electrodes highlighted in black ina, and simulated concentration-versus-diffusion time results at two locations matching the locations of these two electrodes, assuming a diffusion constant of 0.5 × 10−9m2s−1. (e) Simulation of lateral spreading functions from two 1-μm semispherical sources 1 mm apart, for an agar slab thickness of 900 μm and with a diffusion time of 3 min. (f) Lateral resolution versus diffusion time for two 1-μm semi-spherical sources on a 900-μm agar surface, as well as signal-to-noise ratio (SNR) versus diffusion time for three uniform source concentrations on the top surface of the agar film. Figure 4: Characterization of phenazine diffusion. ( a ) Experimental schematic for on-chip diffusion characterization. The pyocyanin (PYO)-soaked piece of membrane is shown in green, whereas the two probed electrodes are highlighted in black. Scale bar, 1 mm. ( b ) Simulation model of the experiment, consisting of a 4 × 4 × 0.9 mm 3 block with a constant 71 μM concentration at the blue surface. ( c ) Simulation results, showing concentration at the bottom surface of the block. ( d ) Experimental concentration-versus-diffusion time results at the two electrodes highlighted in black in a , and simulated concentration-versus-diffusion time results at two locations matching the locations of these two electrodes, assuming a diffusion constant of 0.5 × 10 −9 m 2 s −1 . ( e ) Simulation of lateral spreading functions from two 1-μm semispherical sources 1 mm apart, for an agar slab thickness of 900 μm and with a diffusion time of 3 min. ( f ) Lateral resolution versus diffusion time for two 1-μm semi-spherical sources on a 900-μm agar surface, as well as signal-to-noise ratio (SNR) versus diffusion time for three uniform source concentrations on the top surface of the agar film. Full size image Lateral diffusion in our measurement platform can be understood by solution of the three-dimensional diffusion (heat) equation with a diffusion constant D for molecules originating at a semi-spherical source (of radius a ) on the top surface of an agar slab. The source is assumed to maintain a fixed concentration on its surface. a can be chosen to match typical dimensions of the bacterial cells being studied. Concentrations are observed on the bottom surface of the agar with zero-flux boundary conditions assumed on both the top and bottom of the agar film. Solutions to the diffusion equation can be simulated with finite-element models or solved analytically in some cases (see Supplementary Methods for analytical solution formulations). To analyse the effects of horizontal diffusion on spatial resolution, we consider two semi-spherical sources of radius a =1 μm of the same concentration, a horizontal distance d apart on the top surface of the agar and simulate the concentration at the bottom of the 900-μm thick agar slab as a function of diffusion time ( Fig. 4e ). We define resolution as the minimum horizontal distance d at which two separate peaks can be discriminated. Figure 4f shows the degradation in this lateral resolution with diffusion time. To analyse vertical diffusion, we solve the one-dimensional diffusion equation for a uniform concentration at the top surface of the agar and calculate the concentration at the bottom of the 900-μm thick agar film. Figure 4f shows the resulting SNR for top surface concentrations of 500, 100 and 20 μM as a function of diffusion time (using the maximum noise level shown in Fig. 3f ). As expected, SNR improves over time as more molecules arrive at the bottom of the agar for detection. For our colony experiments, we choose to capture images after a diffusion time of 3 min, at which time SNR will surpass three for concentrations greater than 20 μM and a resolution of 750 μm is expected. 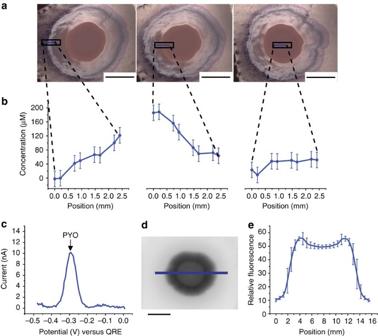Figure 5: On-chip spatially resolved detection of pyocyanin. Shown are results fromP. aeruginosaPA14 wild-type colony biofilms. (a) Regions within colony biofilms that are imaged. The black box represents the field of view of the integrated circuit (IC), and the blue line represents the column of pixels (electrodes) probed. Scale bars, 5 mm. (b) Pyocyanin (PYO) concentration as a function of location for a single imager column within the colony regions that are highlighted ina. Concentrations are determined based on current-to-concentration calibration curves. Error bars represent the measured standard deviation in quantifying concentration based on current-to-concentration calibration curves. (c) Example baseline-subtracted, positive-to-negative square wave voltammogram from a single electrode, showing the PYO peak. QRE, quasireference electrode. (d) Representative fluorescence image from a wild-typeP. aeruginosaPA14 colony with a green fluorescent protein (GFP) reporter under the control of thephzA2promoter. Data along the drawn blue line are plotted ine. Scale bar, 5 mm. (e) Position-dependentphzA2expression. The average fluorescence resulting from thephzA2promoter-driven GFP expression is shown for five colonies. Error bars represent the standard deviation of the five experiments, and are shown for 15% of the data points. Spatially resolved detection of phenazines in biofilms Figure 5a,b shows the electrochemical imaging possible in WT P. aeruginosa PA14 colony biofilms grown under typical experimental conditions. Specifically, we image the PYO concentration after a diffusion time of 3 min using positive-to-negative SWV. PYO concentration profiles that result from three separate images taken at different positions in the colonies ( Fig. 5a ) are plotted in Fig. 5b for one pixel column, with a representative square wave voltammogram from a single electrode shown in Fig. 5c . The error bars in Fig. 5b represent the measured standard deviation in quantifying concentration based on current-to-concentration calibration curves and, therefore, exceed the noise values quantified in Fig. 3f , as this error estimate also includes experiment-to-experiment variability in electrode and agar conditions. The PYO concentration increases towards the edge of the colony. In previously published work, we have shown that in P. aeruginosa PA14 the phzA2-G2 operon is required for biofilm-specific production of phenazines, whereas the nearly identical operon phzA1-G1 does not contribute significantly [24] . Here we follow expression of phzA2 , the first gene of the phzA2-G2 operon, using a green fluorescent protein (GFP) reporter. The phzA2 expression pattern ( Fig. 5a,b ) is consistent with the electrochemically observed PYO distribution along the colony cross-section ( Fig. 5d,e ). Figure 5: On-chip spatially resolved detection of pyocyanin. Shown are results from P. aeruginosa PA14 wild-type colony biofilms. ( a ) Regions within colony biofilms that are imaged. The black box represents the field of view of the integrated circuit (IC), and the blue line represents the column of pixels (electrodes) probed. Scale bars, 5 mm. ( b ) Pyocyanin (PYO) concentration as a function of location for a single imager column within the colony regions that are highlighted in a . Concentrations are determined based on current-to-concentration calibration curves. Error bars represent the measured standard deviation in quantifying concentration based on current-to-concentration calibration curves. ( c ) Example baseline-subtracted, positive-to-negative square wave voltammogram from a single electrode, showing the PYO peak. QRE, quasireference electrode. ( d ) Representative fluorescence image from a wild-type P. aeruginosa PA14 colony with a green fluorescent protein (GFP) reporter under the control of the phzA2 promoter. Data along the drawn blue line are plotted in e . Scale bar, 5 mm. ( e ) Position-dependent phzA2 expression. The average fluorescence resulting from the phzA2 promoter-driven GFP expression is shown for five colonies. Error bars represent the standard deviation of the five experiments, and are shown for 15% of the data points. Full size image Unlike gene expression reporter-based approaches, our IC-based platform technique allows us to distinguish and simultaneously image multiple phenazines directly. We use the P. aeruginosa PA14 mutant strain BigBlue (DKN370) [9] , which overproduces 5-MCA and PYO, and perform on-chip positive-to-negative SWV imaging of the two phenazines at multiple locations within a BigBlue colony biofilm ( Fig. 6a ). 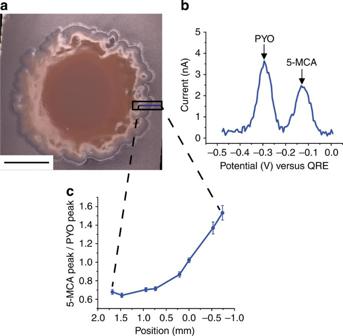Figure 6: On-chip spatially resolved detection of multiple phenazines. Shown are results from aP. aeruginosaPA14 BigBlue9colony biofilm. (a) Region within a BigBlue colony that is electrochemically imaged. The black box represents the field of view of the integrated circuit (IC), and the blue line represents the column of pixels (electrodes) probed. Scale bar, 5 mm. (b) Example baseline-subtracted, positive-to-negative square wave voltammogram from a single electrode, showing the pyocyanin (PYO) and 5-methylphenazine-1-carboxylic acid (5-MCA or a derivative thereof) current peaks analysed. QRE, quasireference electrode. (c) Ratio of 5-MCA to PYO concentration along one pixel column for the imaged region shown ina. Error bars account for noise in the square wave voltammetry (SWV) recordings, using the maximum noise level found inFig. 3f. In calculating the error bars, 5-MCA and PYO currents are assumed to be uncorrelated. Figure 6b shows a representative waveform at a single electrode. In Fig. 6c , we plot the ratio of 5-MCA to PYO peak currents, which assuming equal diffusion constants is equal to the ratio of concentrations, as a function of position. The ratio of 5-MCA to PYO rises towards the edge of the colony biofilm. Figure 6: On-chip spatially resolved detection of multiple phenazines. Shown are results from a P. aeruginosa PA14 BigBlue [9] colony biofilm. ( a ) Region within a BigBlue colony that is electrochemically imaged. The black box represents the field of view of the integrated circuit (IC), and the blue line represents the column of pixels (electrodes) probed. Scale bar, 5 mm. ( b ) Example baseline-subtracted, positive-to-negative square wave voltammogram from a single electrode, showing the pyocyanin (PYO) and 5-methylphenazine-1-carboxylic acid (5-MCA or a derivative thereof) current peaks analysed. QRE, quasireference electrode. ( c ) Ratio of 5-MCA to PYO concentration along one pixel column for the imaged region shown in a . Error bars account for noise in the square wave voltammetry (SWV) recordings, using the maximum noise level found in Fig. 3f . In calculating the error bars, 5-MCA and PYO currents are assumed to be uncorrelated. Full size image Distribution of metabolites in multicellular structures is frequently inferred from fluorescent reporter gene expression [25] . Although reporters can be used to monitor expression at both the transcriptional and the translational levels, they cannot assess the activity of the gene product. In the case of phenazine synthesis in P. aeruginosa PA14 colonies, expression patterns of a fluorescent reporter representing the phzA2-G2 operon do not provide information about the specific phenazines produced and are a leading, rather than direct, indicator of actual phenazine production. An alternative method for detecting certain metabolites such as phenazines in vivo is two-photon excitation microscopy, although this method has only been demonstrated on cells in planktonic cultures [14] . Measurements from two-photon excitation microscopy experiments consist of the summed fluorescence signals from the various fluorescent species produced by the bacteria. This total signal must then be decomposed into the component signals from each autofluorescent species using statistical techniques. In contrast, our electrochemical technique naturally results in well-resolved signals from individual phenazines. A further problem is that in aerobic conditions, the fluorescent signal from the WT culture is nearly identical to the signal from a phenazine-null culture because the signal from non-phenazine fluorescent metabolites, present in both cultures, is much stronger than the signal from phenazines due to their low quantum yield. Various mass spectrometry (MS) techniques have been applied to imaging applications in colony biofilms [26] . Although MS techniques show promise for microbial research, they require MS instrumentation generally weighing more than 500 kg and costing in excess of $100,000. MS techniques focus on probing bacterial colony top surfaces, which requires various forms of colony treatment such as liquid bridges [27] , imprinting on a substrate [28] , coating with an organic matrix [29] or incorporation of tags [30] . Our electrochemical platform, which focuses on detecting redox-active species released from the bottom surface of colonies, is capable of detecting molecules from undisturbed films. We must contend with diffusion effects, however, leading to coarser resolutions than the 10–100 μm resolution typically achieved in most MS approaches [26] . Our platform is capable of quantifying the species sensed, which is currently not possible with most MS techniques [26] . Electrochemical detection of phenazines from liquid cultures of P. aeruginosa has been well established using various methods, including adsorptive stripping voltammetry [16] , differential pulse voltammetry [17] , [19] and SWV [18] . Scanning electrochemical microscopy approaches have also been used [20] but cannot be effectively combined with voltage sweep techniques such as adsorptive stripping voltammetry, differential pulse voltammetry and SWV for applications requiring quantification of concentration or detection of multiple species because of prohibitively long analysis times. During the time required to record the image in scanning approaches (up to minutes), significant changes can occur in the biofilm. To achieve fast imaging speed, scanning approaches generally maintain the probe at a constant potential and, therefore, are unable to quantify concentration or to detect multiple species. Key to the methods developed in this work is the exploitation of IC technology as a new tool for biology, enabling many measurement channels and electrodes to be fabricated within a very small area. Integrated microelectronics can enable localized, multiplexed [5] and high-speed [31] recordings not possible with macroscale electrochemical instruments. Cells mediate their physiological activities using secreted molecules. Phenazines are secreted metabolites that control gene expression and alter the intracellular redox state [11] , [32] , [33] . Both phenazine functions are concentration-dependent and are critical in modulating cellular activities during P. aeruginosa PA14 colony biofilm development [9] , [11] . In this study, we report that the colonies produce a phenazine gradient ( Figs 5b and 6c ), which is likely to be of physiological significance and contribute to colony morphogenesis. Pairing genetic manipulation with direct detection of phenazines will allow us to dissect the organizational functions of phenazines further. The studies in this paper also translate to eukaryotes, in which morphogen gradients pattern cells within developmental fields of multicellular structures by means of concentration-dependent signalling relays [34] . Metabolites reflect the physiological states of producing cells. Many metabolites other than phenazines, such as hydrogen peroxide, nitric oxide and sulfide, also have a role in the development of biofilms and eukaryotic tissues. For example, nitric oxide has been implicated in dispersal events of biofilms [35] and is a potent vasodilator [36] . Previous studies have demonstrated that a wide variety of macromolecules and metabolites, including DNA [37] , small molecules [38] , [39] and neurotransmitters [40] , are amenable to electrochemical characterization and, therefore, are suitable for study with the platform developed here. (See Supplementary Figs 5 and 6 for on-chip experiments with other redox-active metabolites.) IC design The chip is a custom IC implemented using a commercial Taiwan Semiconductor Manufacturing Company 0.25 μm CMOS process. The chip was designed and simulated using the Cadence Virtuoso software package (Cadence; see Supplementary Figs 7–10 and Supplementary Methods for circuit design details). Electrode modifications The working electrodes were initially implemented in aluminium, the top metal layer of the CMOS process. These electrodes were converted to gold using the following process. Photoresist (AZ Electronic Materials, AZ4620) was spun onto the chip using a two-step programme of 300 r.p.m. for 3 s and 4,500 r.p.m. for 45 s, followed by a soft bake at 110 °C for 2 min. The chip was exposed at 6.8 mW cm −2 for 35 s in a mask aligner (SUSS MA6) using a chrome-on-glass mask that defines openings above the working electrodes. For development, the chip was immersed in a 1:3 mixture of developer (AZ Electronic Materials, AZ400K) and water for approximately 90 s. The exposed aluminium was etched in heated aluminium etchant (Transene Aluminum Etchant Type A) for 5 min. Titanium/gold of 4 nm/135 nm thickness was evaporated onto the chip in an electron beam evaporator (Semicore SC2000), followed by lift-off in acetone. Packaging and supporting electronics The die was wire bonded to a 272-pin ball-grid-array package. Dam-and-fill doughnut epoxy encapsulation (Hysol FP4451 dam and FP4650 fill) covered the exposed gold wire bonds, leaving the die surface exposed. The chip was then mounted on a circuit board containing power supply circuitry, a digital-to-analog converter operating at 2 kHz for inputting the voltage signal during measurements, an anti-aliasing filtre with a 1-kHz cutoff, an analog-to-digital converter operating at 13 kHz for converting the TIA outputs during measurements, and a field-programmable gate array module (Opal Kelly XEM3010) with a Universal Serial Bus interface for the transfer of digital signals to and from the chip and printed circuit board (see Supplementary Fig. 11 ). Square wave voltammogram processing The output current signal from a SWV experiment consisted of the response to a series of forward and reverse voltage steps. To create the square wave voltammogram, the current value at the end of each voltage step was sampled. Pairs of consecutive current samples, one after a forward voltage step and one after a reverse voltage step, were subtracted from each other. In on-chip SWV experiments, the six current values at the end of each voltage step were averaged together (rather than just using the final current value) to counter noise. The resulting signal was plotted as a function of applied potentiostat voltage. For quantification of peak heights, the peak current was measured from a baseline, which was taken to be the square wave voltammogram measured on pure agar at the same applied voltage. CMOS chip electrochemical measurements On-chip electrochemical cells consisted of an on-chip gold working electrode, an external platinum counter electrode and an external chlorinated silver wire serving as a QRE in a three-electrode potentiostat configuration. The feedback loop established the excitation voltage signal on the reference electrode. The working electrode was maintained at a constant potential and was connected to a TIA to read the output current. The SWV excitation signal consisted of a staircase ramp with 6 mV increments, 25 mV staircase amplitude and 50 Hz frequency. (See Supplementary Figs 12 and 13 and Supplementary Methods for a discussion of the effects of SWV frequency on signal-to-noise performance.) The voltage range of the input signal was either from −0.5 or −0.7 V to 0 V. The TIA was set to a gain of 10 MΩ. For each colony measurement, the chip was covered with an agar layer (1% agar, 1% tryptone), approximately 1 mm thick. A piece of track-etched membrane (Whatman 111707, pore size=0.4 μm) with a biofilm growing on top was transferred onto the agar layer. The external counter and QRE were embedded in the agar layer as well. After 3 min, square wave voltammograms were measured at eight electrodes from a single column in the IC’s electrode, one after another. Total measurement time for all eight electrodes was 64 s. CMOS chip calibration To perform concentration calibration, known concentrations of phenazines solvated in agar were measured. Concentrated solutions of phenazines were prepared by allowing P. aeruginosa PA14 to grow on agar for weeks, until the phenazine concentration in the agar was hundreds of micromolar. Calibration curves were constructed for each on-chip electrode by measuring the peak current on square wave voltammograms from a series of diluted solutions of the concentrated agar. Phenazines in the agar were separated and quantified as described below. Potentiostat electrochemical measurements For comparison, electrochemical measurements of synthetic phenazines and agar extracts were also taken using a commercial potentiostat (CH Instruments, CHI760D) with an electrochemical cell consisting of a 1.6-mm-diameter gold working electrode, a platinum counter electrode and a Ag/AgCl reference electrode (BASI). The SWV input signal consisted of a staircase ramp between −0.8 and 0.2 V in both directions, with 10 mV increments, 50 mV stair amplitude and 10 Hz frequency. (See Supplementary Fig. 1 and Supplementary Methods for a further discussion of the effects of frequency.) Preparation of colonies Liquid cultures were grown in lysogeny broth [41] at 37 °C with shaking at 250 r.p.m. overnight. Colonies used for phenazine extractions were grown on solid medium containing 1% agar and 1% tryptone [24] . Colonies used for on-chip electrochemical measurements were prepared by spotting 10 μl of a cell suspension onto a track-etched membrane (Whatman 111707, pore size=0.4 μm) placed upon a 1% agar, 1% tryptone plate containing 40 μg ml −1 Congo red and 20 μg ml −1 Coomassie blue. The colonies were grown at 25 °C, >95% humidity for the desired time and then imaged using a digital microscope (Keyence, VHX-1000). Supplementary Table 1 lists the strains used in this study. Preparation and quantification of agar extracts Agar extracts were prepared for phenazine quantification and electrochemical detection of phenazine derivatives. Four 100 μl droplets of a cell suspension were spotted onto agar plates containing 40 ml of 1% agar, 1% tryptone and grown for 1 day. Phenazines were extracted from the agar by scraping off the colonies with a razor blade and soaking the agar in 3 ml of phosphate-buffered saline overnight. The extract was then collected and stored at 4 °C. For electrochemical detection of synthetic and purified phenazine derivatives, extract from Δ phz colonies was used as solvent. Phenazines were separated and quantified from filtered (0.2 μm pore) agar extracts using high-performance liquid chromatography. Fifty microlitres of sample was loaded onto an analytical Waters Symmetry C-18 reverse phase column (Waters; 5 μm particle size, 4.6 × 150 mm 2 ). The phenazines were separated using a gradient of water-0.01% TFA (solvent A) to acetonitrile-0.01% TFA (solvent B) at a flow rate of 0.6 ml min −1 using the following protocol: linear gradient from 0 to 15% solvent B for 2 min, linear gradient to 83% solvent B for 20 min, linear gradient from 83 to 100% solvent B for 10 min and finally, a linear gradient to 0% solvent B for 5 min. The total method time was 38 min. The retention times for PYO, PCN and PCA were 10 min, 17 min and 20 min, respectively. The concentration of each phenazine species was determined by taking the area under each peak using System Gold 32 Karat Software (Beckman Coulter) with the following conversion factors: 8 × 10 6 μM AU −1 for PYO and 9.5 × 10 6 μM AU −1 for PCN and PCA. Phenazine solutions Synthetic PYO (Cayman Chemical) was diluted to 10 μM in agar extract from Δ phz colonies. Synthetic PCA (Princeton Biomolecular Research) was diluted to 300 μM in Δ phz agar extract. PCN purification Four 100 μl colonies were spotted on 11 1% agar, 1% tryptone plates. 700 μl was spread onto 12 additional 1% agar, 1% tryptone plates using glass beads. The cultures were grown at 25 °C and >95% humidity for 5 days. The colonies were scraped from the agar using a razor blade, and the agar was added to a 2-l flask. Phenazines were extracted by soaking the agar in 400 ml of PBS, pH 7.4 overnight (light-protected and at room temperature). The extract was centrifuged at 4,500 r.p.m. for 5 min. The supernatant was extracted using an equal volume of chloroform, and the organic phase was recovered and rotovapped to dryness. 400 μl of methanol was added to the dried extract, and this solution was filtered through a 0.22-μm filtre. 200 μl of this solution was loaded onto a preparative Waters Sun Fire C-18 reverse column (Waters; 5-μm particle size, 19 × 100 mm column). The phenazines were separated using water with 0.01% TFA (solvent A) and acetonitrile with 0.01% TFA (solvent B) at a flow rate of 1.0 ml min −1 using the following protocol: linear gradient 0–15% solvent B for 2 min, linear gradient 15–83% solvent B for 20 min, linear gradient from 83 to 100% solvent B for 15 min, 100% solvent B for 15 min and finally, linear gradient from 100 to 0% solvent B for 2 min. The entire method time was 58.5 min. The retention time of PCN was 37.8 min. Twenty fractions were collected in 1 min increments. The OD 366 of each fraction was measured to identify samples containing PCN. This sample was rotovapped to dryness and dried for 15 min using a vacuum. The powder was resuspended in 2 ml of Δ phz agar extract giving a final PCN concentration of 3 mM. Quantification of fluorescent reporters Ten microlitres of overnight cultures of WT P phzA2- GFP (see Supplementary Tables 1 and 2 ) were spotted onto a track-etched membrane with 0.4 μm pore size (Whatman 111707) placed atop 1% agar, 1% tryptone plates containing 20 μg ml −1 Coomassie blue and 40 μg ml −1 Congo red. The colonies were grown for 2 days and imaged using a Typhoon scanner (GE Healthcare). The excitation wavelength was 488 nm and the emission was measured at 520 nm. The images were processed using surface plot analysis in ImageJ ( http://imagej.nih.gov/ij/ ). Diffusion modeling Simulations were performed in COMSOL using the Transport-of-Dilute-Species feature. The diffusion coefficient of the chemical species was set at 0.5 × 10 −9 m 2 s −1 . Initial concentrations in all non-source areas were set to zero, and no-flux conditions were enforced at all the surfaces of the block. How to cite this article: Bellin, D. L. et al . Integrated circuit-based electrochemical sensor for spatially resolved detection of redox-active metabolites in biofilms. Nat. Commun. 5:3256 doi: 10.1038/ncomms4256 (2014).